Inducing effect on the percolation transition in complex networks Percolation theory concerns the emergence of connected clusters that percolate through a networked system. Previous studies ignored the effect that a node outside the percolating cluster may actively induce its inside neighbours to exit the percolating cluster. Here we study this inducing effect on the classical site percolation and K -core percolation, showing that the inducing effect always causes a discontinuous percolation transition. We precisely predict the percolation threshold and core size for uncorrelated random networks with arbitrary degree distributions. For low-dimensional lattices the percolation threshold fluctuates considerably over realizations, yet we can still predict the core size once the percolation occurs. The core sizes of real-world networks can also be well predicted using degree distribution as the only input. Our work therefore provides a theoretical framework for quantitatively understanding discontinuous breakdown phenomena in various complex systems. Percolation transition on complex networks occurs in a wide range of natural, technological and socioeconomic systems [1] , [2] , [3] . The emergence of macroscopic network connectedness, due to either gradual addition or recursive removal of nodes or links, can be related to many fundamental network properties, for example, robustness and resilience [4] , [5] , cascading failure [3] , [6] , [7] , epidemic or information spreading [8] , [9] and structural controllability [11] , [12] . Particularly interesting are the emergence of a giant connected component [13] , [14] , [15] , [16] , [17] , [18] , [19] , [20] , [21] , the K -core (obtained by recursively removing nodes with degree less than K ) [22] , [23] , [24] , [25] , and the core (obtained by recursively removing nodes of degree one and their neighbours) [12] , [26] , [27] . These classical percolation processes are passive in the sense that whether or not a node belongs to the percolating cluster depends only on its number of links to the percolating cluster. However, in many physical or information systems, each node has an intrinsic state and after a node updates its state, it can actively induce its neighbours to update their states too. One example is the frozen-core formation in Boolean satisfiability problems [28] , where non-frozen nodes can induce its frozen neighbours into the non-frozen state (the so-called whitening process [29] , [30] , [31] ). In the glassy dynamics of kinetically constrained models, a spin in a certain state facilitates the flipping of its neighbouring spins [32] . In inter-dependent networks, a collapsed node of one network causes the failure of the connected dependent node in the other network [3] , [33] , resulting in a damage cascading process. The inducing effect can also be related to information or opinion spreading, for example, an early adopter of a new product or innovation might persuade his or her friends to adopt either. Despite its implications on a wide range of important problems, the inducing effect on percolation transitions has not been fully understood. In this work, we study the inducing effect on the classical site percolation and K -core percolation in complex networks. We analytically show that the inducing effect always causes a discontinuous percolation transition, therefore providing a new perspective on abrupt breakdown phenomena in complex networked systems. Our analytical calculations are confirmed by extensive numerical simulations. Description of the model We assume each node of the network has a binary internal state: protected or unprotected. We allow an initial p fraction of nodes randomly chosen from the network to be protected. If p =1, all the nodes are initially protected. As time evolves, a protected node spontaneously becomes unprotected if it has less than K protected neighbours. (In case of K =0, a protected node will never spontaneously become unprotected.) A protected node with K or more protected neighbours will be induced to the unprotected state if at least one of its unprotected neighbours has less than K ′ protected neighbours. (In case of K ′=0 or 1, the inducing effect is absent and our model reduces to the classical site percolation or K -core percolation.) Note that once a node becomes unprotected it will remain unprotected. We refer to the above-mentioned evolution process as the ( K , K ′)-protected core percolation. The ( K , K ′)-protected core, or simply, the protected core is the subnetwork formed by all the surviving protected nodes and the links among them (see Fig. 1 for an example). We denote the total number of nodes in the protected core as N p-core . We can prove that the protected core is independent of the particular state evolution trajectory of the nodes and hence is well defined (see Supplementary Note 1 ). 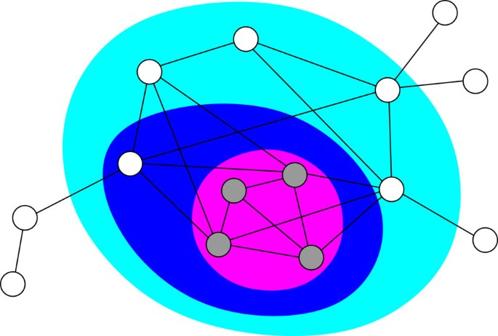Figure 1: The (2,2)-protected core of a small network. The (2,2)-protected core (magenta region) is contained in the core (blue), which is then contained in the 2-core (cyan). Protected and unprotected nodes are coloured in gray and white, respectively. Figure 1: The (2,2)-protected core of a small network. The (2,2)-protected core (magenta region) is contained in the core (blue), which is then contained in the 2-core (cyan). Protected and unprotected nodes are coloured in gray and white, respectively. Full size image In the context of opinion spreading or viral marketing, the ( K , K ′)-protected core percolation can be described as follows: consider a population of users to adopt a new product (or idea, opinion, innovation and so on). Initially there is a p fraction of users in the ‘protected’ (or conservative) state and refuse to adopt the new product. The other (1– p ) fraction of users are in the ‘unprotected’ state, that is, they are early adopters. A conservative user will automatically adopt the new product if he/she has less than K conservative friends. An adopted user with less than K ′ conservative friends will persuade all his or her conservative friends to adopt the new product. Then the protected core, if exists, can be viewed as the subnetwork of the most conservative individuals, who will never adopt the new product. Analytical approach Consider a large uncorrelated random network containing N nodes, with arbitrary degree distribution P ( k ) and mean degree [34] , [35] . We assume that if any node i is still in the protected state, its neighbours do not mutually influence each other and therefore their states are independently distributed. This is a slight extension of the Bethe–Peierls approximation widely used in spin-glass theory and statistical inference [36] . Note that a closely related approximation in network science is the tree approximation [5] , [14] , [34] , which assumes the neighbours of node i become disconnected if i is removed from the network. Under our assumption of state independence, we can calculate the normalized size n p-core (≡ N p-core / N ) of the protected core as with being the binomial coefficient (see Supplementary Note 2 ). The parameter α denotes the probability that, starting from a node i that is still in the protected state, a node j reached by following a randomly chosen link ( i , j ) is in the unprotected state and having at most K ′–1 protected neighbours (including i ). The parameter β is the probability that such a node j is in the unprotected state but having at least K ′ protected neighbours. We further define γ as the probability that such a node j is in the protected state and having exactly K protected neighbours. Note that if initially we randomly choose a finite p fraction of nodes to be protected, then (1– p ) fraction of the nodes will be and remain unprotected. Let us define η as the probability that, starting from such an initially unprotected node m , a node n reached by following a randomly chosen link ( m , n ) will eventually be in the unprotected state even if the inducing effect of node m is not considered. Because of the inducing effect, each node j mediates strong correlations among the states of its neighbouring nodes if it is in the unprotected state. After a careful analysis of all the possible microscopic inducing patterns following the theoretical method of Zhou [37] , [38] , we obtain a set of self-consistent equations for the probabilities α , β , γ and η : where Q ( k ) ≡ kP ( k )/ c is the degree distribution for the node at an end of a randomly chosen link. These equations can be understood as follows. The first term on the right hand side of Equation (2) is the probability that a node j reached by following a link ( i , j ) is initially unprotected and having at most K ′–2 protected neighbours (excluding node i ) without considering its inducing effect. The other two terms in the right hand side of Equation (2) yield the probability that an initially protected node j at the end of a link ( i , j ) will either spontaneously transit to or be induced to the unprotected state and, when it is still in the protected state, at most K ′–2 of its protected neighbours (excluding node i ) have more than K protected neighbours themselves. The terms in Equations (3)–(5), can be understood similarly (see Supplementary Note 2 for more explanations). The above self-consistent equations can be solved using a simple iterative scheme (see Supplementary Note 3 ). When K , K ′ ≥ 2, these equations always have a trivial solution ( α , β , γ , η )=(1,0,0,1), yielding no protected core ( n p-core =0). This solution is always locally stable, and it is the only solution if the mean degree c of the network is small or the initial fraction p of protected nodes is small (see Supplementary Note 4 ). As c (or p ) increases, another stable solution of Equations (2)–(5) appears at the critical mean degree c = c * (or the critical fraction p = p *), corresponding to the percolation transition. In the limiting cases of K ε{0,1}, Equations (2)–(5), also change from having only one stable solution to having two distinctive stable solutions at certain critical value c = c * or p = p * (see Supplementary Note 4 ). The minimal inducing effect The minimal inducing effect on percolation transitions can be demonstrated by comparing (0,1)- and (1,1)-protected core percolation transitions with (0,2)- and (1,2)-protected core percolation transitions as we tune the initial fraction of protected node p . Note that the ( K ,1)-protected core percolation with K ε{0,1} is essentially the classical site percolation [1] , [5] , [14] , because a protected node will remain protected if it has at least one protected neighbour and there is no inducing effect at all. In this case, a giant connected component of protected nodes gradually emerges in the network as p exceeds (see Fig. 2 ). The minimal inducing effect is naturally present in the (0,2)- and (1,2)-protected core percolation problems, namely if an unprotected node has only one protected neighbour, this neighbour will be induced to the unprotected state. In this case our analytical calculation shows that both the normalized size of the protected core and that of its giant connected component will jump from zero to a finite positive value at certain critical value p * (see Supplementary Notes 4 and 5 ). For Erdös–Rényi (ER) random networks [39] , [40] with mean degree c =10, this threshold fraction is p *≈0.44 (for K =1) and p *≈0.42 (for K =0), which are much larger than the threshold value p *=0.1 of the classical continuous site percolation transition (see Fig. 2 ). Note that in case K =0, a protected node will never spontaneously become unprotected, hence the discontinuous (0,2)-protected core percolation transition is solely due to the inducing effect. 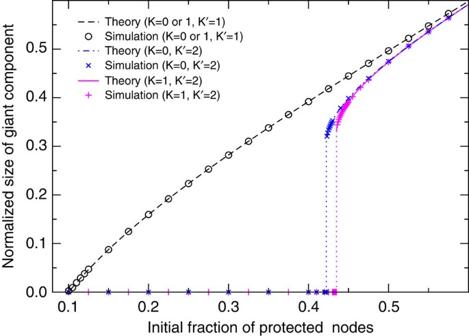Figure 2: Size of giant connected component of protected nodes. Symbols are simulation results on a single ER random network ofN=106nodes and mean degreec=10, whereas the lines are theoretical predictions atN=∞. The giant connected component of protected nodes continuously emerges in the (0,1)- and (1,1)-protected core percolation problems (without inducing effect), but it emerges discontinuously in the (0,2)- and (1,2)-protected core percolation problems (with minimal inducing effect). Figure 2: Size of giant connected component of protected nodes. Symbols are simulation results on a single ER random network of N =10 6 nodes and mean degree c =10, whereas the lines are theoretical predictions at N =∞. The giant connected component of protected nodes continuously emerges in the (0,1)- and (1,1)-protected core percolation problems (without inducing effect), but it emerges discontinuously in the (0,2)- and (1,2)-protected core percolation problems (with minimal inducing effect). Full size image Inducing effect on K -core percolation The inducing effect can also be demonstrated by comparing the K -core percolation and the ( K , K ′)-protected core percolation as we tune the mean degree c . In the following discussions, we set p =1 and focus on the representative case of K ′= K (the results for p <1 and 2≤ K ′≠ K are qualitatively the same). And we refer to ( K , K )-protected core simply as K -protected core. We find that for any K≥ 2, as c reaches the critical value c *, n p-core jumps from zero to a finite value (see Supplementary Note 4 ), indicating a discontinuous percolation transition. We also find that for any K≥ 2 and independent of network types, in the supercritical regime where c – c *→0 + (see Supplementary Note 6 ). Such a hybrid phase transition and the associated critical exponent 1/2 were also observed in K -core percolation and core percolation [12] , [22] , [23] , [24] . In the following, we study the discontinuous 2-protected core percolation in a series of random networks with specific degree distributions. We first consider the ER random network with Poisson degree distribution P ( k )= e − c c k / k !. We find that the discontinuous 2-protected core percolation transition occurs at c = c *≈3.92, with a jump of n p-core from zero to (see Fig. 3 ). Note that for ER random networks the classical 2-core and core percolation transitions occur at c *=1 and c *= e ≈2.72, respectively, and they are both continuous [12] , [24] . Hence, allowing unprotected nodes to induce other nodes not only delays the occurrence of the percolation transition to a larger value of c but also makes it discontinuous (see Fig. 4 ). 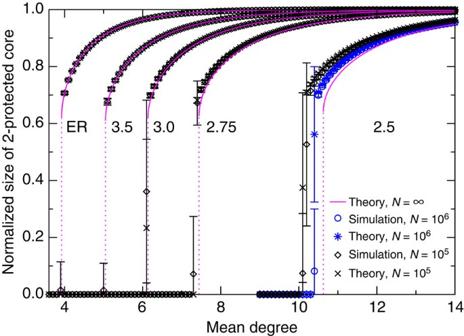Figure 3: Size of 2-protected core for ER networks and SF networks. The degree exponents of the SF networks areλ=3.5,3.0,2.75,2.5 (from left to right). Lines are analytic predictions for infinite system (N=∞), circles and diamonds are exact results obtained through the state evolution process; star and cross symbols are the analytic results using the exact degree sequences of the constructed networks. Each simulation point is obtained by averaging over 80 independent network instances. Note that forλ<3, especially whenλ→2, significant finite-size effect is observed. This is rooted in the intrinsic degree correlations in the static model whenλ<341,42,43. Figure 3: Size of 2-protected core for ER networks and SF networks. The degree exponents of the SF networks are λ =3.5,3.0,2.75,2.5 (from left to right). Lines are analytic predictions for infinite system ( N =∞), circles and diamonds are exact results obtained through the state evolution process; star and cross symbols are the analytic results using the exact degree sequences of the constructed networks. Each simulation point is obtained by averaging over 80 independent network instances. Note that for λ <3, especially when λ →2, significant finite-size effect is observed. This is rooted in the intrinsic degree correlations in the static model when λ <3 [41] , [42] , [43] . 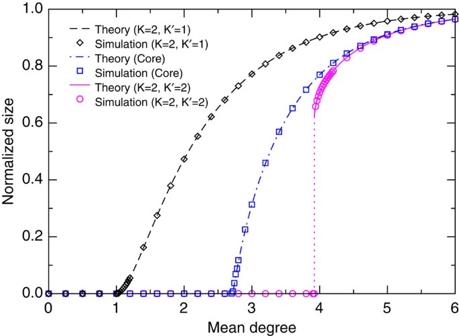Figure 4: Comparing the percolation transitions. Symbols are simulation results on a single ER random network ofN=106nodes, whereas the lines are theoretical predictions atN=∞. Both the 2-core (equivalent to the (2,1)-protected core) and the core emerges continuously but the 2-protected core emerges discontinuously. Full size image Figure 4: Comparing the percolation transitions. Symbols are simulation results on a single ER random network of N =10 6 nodes, whereas the lines are theoretical predictions at N =∞. Both the 2-core (equivalent to the (2,1)-protected core) and the core emerges continuously but the 2-protected core emerges discontinuously. Full size image Scale-free (SF) networks characterized by a power-law degree distribution with degree exponent λ are ubiquitous in real-world complex systems [39] . Interestingly, we find that for purely scale-free networks with P ( k )= k − λ / ζ ( λ ) and ζ ( λ ) the Riemann ζ function, the K -protected core does not exist for any λ >2 (see Supplementary Note 7 ). If the smallest degree k min ≥K and a fraction ρ of the links are randomly removed from the purely SF network, then a discontinuous K -protected core percolation transition will occur (see Supplementary Note 7 ). For asymptotically SF networks generated by the static model with for large k only [41] , [42] , [43] , the K -protected core develops when the mean degree c exceeds a threshold value c *. For this type of random networks with different values of c and λ , we compare the theoretical and simulation results and find that they agree well with each other (see Fig. 3 ). For random regular networks, all the nodes have the same degree k 0 , and the K -protected core contains the whole network when k 0 ≥ K . If a randomly chosen fraction ρ of the links are removed, the degree distribution of the diluted network is given by with mean degree c =(1– ρ ) k 0 . We predict that (for k 0 =4) and (for k 0 =6) at the 2-protected core percolation transition, with c *≈3.08 and c *≈3.37, respectively. These predictions are in full agreement with simulation results (see Fig. 5 ). 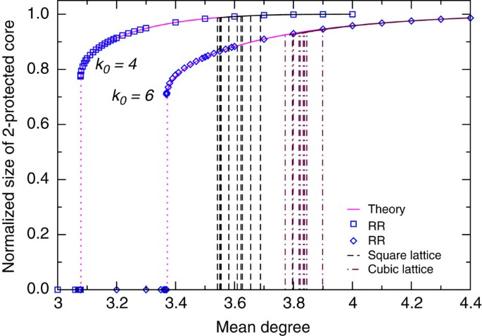Figure 5: Size of 2-protected core for RR networks and regular lattices. Solid and dotted lines are analytic predictions for infinite system. Squares and diamonds are simulation results obtained on a diluted RR network instance with node degreek0=4 andk0=6, respectively, whereas dashed and long-dashed lines are the simulation results obtained on 20 independent diluted network instances of the square and cubic lattice. Each simulated network hasN=106nodes. Figure 5: Size of 2-protected core for RR networks and regular lattices. Solid and dotted lines are analytic predictions for infinite system. Squares and diamonds are simulation results obtained on a diluted RR network instance with node degree k 0 =4 and k 0 =6, respectively, whereas dashed and long-dashed lines are the simulation results obtained on 20 independent diluted network instances of the square and cubic lattice. Each simulated network has N =10 6 nodes. Full size image We also study the 2-protected core percolation in diluted D -dimensional hypercubic lattice and again find a discontinuous transition. Interestingly, in low dimensions the numerically observed transition point c * is remarkably larger than the theoretical prediction (see Figs 5 and 6 ). We find that this difference is not a finite-size effect but intrinsic (it remains in the N →∞ limit), and the difference decreases quickly as D increases. The transition point c * fluctuates considerably for low dimensions (especially for D =2,3) and depends considerably on the system size N (for D ≤7, see Supplementary Note 8 ). Moreover, there is no critical scaling behaviour in the supercritical regime (similar absence of critical scaling was also observed in 4-core percolation on D =4 lattices [44] ). Surprisingly, the value of n p-core at and after the percolation transition agrees well with our theoretical prediction (see Fig. 5 ). 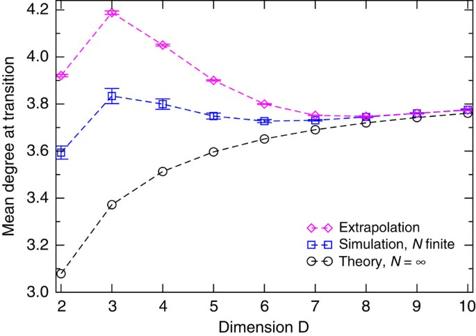Figure 6: 2-protected core percolation point for hypercubic lattice. Each square is the value of the percolation transition point,c*, obtained for aD-dimensional lattice by averaging over 1,600 independent diluted network instances withN2 × 106nodes, diamonds are extrapolated simulation results toN=∞, and circles are analytical predictions ofc* for an infinite RR network with vertex degreek0=2D. The differences between the extrapolated simulation results and the theoretical predictions are due to the ignorance of lattice structures in the theory. Figure 6: 2-protected core percolation point for hypercubic lattice. Each square is the value of the percolation transition point, c *, obtained for a D -dimensional lattice by averaging over 1,600 independent diluted network instances with N 2 × 10 6 nodes, diamonds are extrapolated simulation results to N =∞, and circles are analytical predictions of c * for an infinite RR network with vertex degree k 0 =2 D . The differences between the extrapolated simulation results and the theoretical predictions are due to the ignorance of lattice structures in the theory. Full size image Finally, we apply our theory to a wide range of real-world networks of different sizes and topologies, and find that for most of these networks the normalized sizes of the 2-protected core can be precisely predicted using the degree distribution as the only input (see Supplementary Tables S1 and S2 and Supplementary Note 9 ). Inducing effect has an important role in many complex networked systems. Yet, little was known about how it will affect classical percolation transitions in complex networks. Here we develop analytical tools to address this problem for arbitrary network topologies. Our key finding, that the local inducing effect causes discontinuous site percolation and K -core percolation (for any K≥ 1), suggests a simple local mechanism to better understand and ultimately predict many abrupt breakdown phenomena observed in various systems, for example, the global failure of a national-wide power grid, the sudden collapse of a governmental system or a network of financial institutions. The results presented here also raise a number of questions, answers to which could further deepen our understanding of complex networked systems. First of all, we can improve the local inducing mechanism to be more realistic, for example, by considering that the parameters K and K ′ might be different for different nodes, an unprotected node may only be able to induce some particular neighbours (for example, in a directed network), or an unprotected node may recover to the protected state with certain rate and so on. Second, for low-dimensional lattice systems, the lattice structures and the associated short loops cause strong local and long-range correlations among the states of the nodes, which should be properly considered in a future refined theory, for example, by changing the form of Q ( k ) to include local degree–degree correlations and by exactly computing the effects of short loops up to certain length. Finally, an interesting optimization problem consists of identifying a minimal set of nodes such that perturbing these nodes to the unprotected state will cause the protected core of the whole network to breakdown. In the context of opinion dynamics or viral marketing, this amounts to identifying a minimal set of users for targeted advertisement so that we can dissolve the protected core and eventually all the users will adopt the new opinion or product. We hope our work will stimulate further research efforts on these and other related interesting and challenging questions. How to cite this article: Zhao, J.-H. et al . Inducing effect on the percolation transition in complex networks. Nat. Commun. 4:2412 doi: 10.1038/ncomms3412 (2013).